Molecular mechanism for 3:1 subunit stoichiometry of rod cyclic nucleotide-gated ion channels Molecular determinants of ion channel tetramerization are well characterized, but those involved in heteromeric channel assembly are less clearly understood. The heteromeric composition of native channels is often precisely controlled. Cyclic nucleotide-gated (CNG) channels from rod photoreceptors exhibit a 3:1 stoichiometry of CNGA1 and CNGB1 subunits that tunes the channels for their specialized role in phototransduction. Here we show, using electrophysiology, fluorescence, biochemistry, and X-ray crystallography, that the mechanism for this controlled assembly is the formation of a parallel 3-helix coiled-coil domain of the carboxy-terminal leucine zipper region of CNGA1 subunits, constraining the channel to contain three CNGA1 subunits, followed by preferential incorporation of a single CNGB1 subunit. Deletion of the carboxy-terminal leucine zipper domain relaxed the constraint and permitted multiple CNGB1 subunits in the channel. The X-ray crystal structures of the parallel 3-helix coiled-coil domains of CNGA1 and CNGA3 subunits were similar, suggesting that a similar mechanism controls the stoichiometry of cone CNG channels. The precise assembly of many ion channels relies on a multimerization domain that assembles compatible subunits and excludes incompatible subunits. In the voltage-gated family of channels, these multimerization domains take the form of either an amino-terminal tetramerization domain (T1 domain) [1] , [2] or a carboxy-terminal four helix coiled-coil domain [3] , [4] , [5] . Although channel assembly is generally permitted without these multimerization domains, such domains confer subunit-specific assembly, often restricting the channel composition to like-subunits. Cyclic nucleotide-gated (CNG) channels, however, have a more complex subunit composition. Native CNG channels are composed of a stereotyped number of CNGA subunits and CNGB subunits. CNGA and CNGB subunits are structurally related and both are thought to contribute to the formation of the pore. The CNG channel from rod photoreceptors is composed of three CNGA1 subunits and one CNGB1 subunit [6] , [7] , [8] , whereas the CNG channel from olfactory receptors is composed of two CNGA2 subunits, one CNGA4 subunit and one CNGB1b subunit [9] . The cone CNG channels comprise CNGA3 subunits and CNGB3 subunits, though the subunit stoichiometry is still unknown [8] , [10] . The presence of the CNGB subunits confers enhanced Ca 2+ permeation, modulation by Ca 2+ -calmodulin, and native-like cyclic-nucleotide specificity compared with homomeric CNGA channels [11] , [12] , [13] , [14] , [15] , [16] , [17] . The precisely controlled subunit compositions, therefore, tune the CNG channels for their specialized roles in phototransduction and olfactory transduction. CNG channels are activated by the direct binding of intracellular cyclic nucleotides [18] . They are members of the voltage-gated ion channel superfamily, consisting of four subunits around a centrally located pore. The intracellular carboxy-terminal region of each subunit consists of a C-linker region, a cyclic nucleotide-binding domain (CNBD), and a post-CNBD region ( Fig. 1a ). The X-ray crystal structure of the carboxy-terminal region of the related hyperpolarization-activated cyclic nucleotide-gated channel reveals a four fold symmetric tetramer with non-interacting CNBDs and extensive intersubunit interactions between C-linker regions [19] . 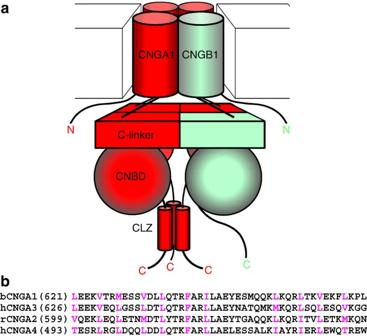Figure 1: Heteromeric rod CNG channel. (a) Cartoon of the heteromeric rod CNG channel composed of three CNGA1 subunits (red) and one CNGB1 subunit (green). The intracellular carboxy-terminal domain contains a C-linker, CNBD, and CLZ domain (only on the CNGA subunits). (b) Sequence alignment of CLZ domains of the different CNGA subunits from bovine (b), rat (r) and human (h). Residues predicted to lie in the 'a' and 'd' positions of heptad repeats are shown in magenta. Figure 1: Heteromeric rod CNG channel. ( a ) Cartoon of the heteromeric rod CNG channel composed of three CNGA1 subunits (red) and one CNGB1 subunit (green). The intracellular carboxy-terminal domain contains a C-linker, CNBD, and CLZ domain (only on the CNGA subunits). ( b ) Sequence alignment of CLZ domains of the different CNGA subunits from bovine (b), rat (r) and human (h). Residues predicted to lie in the 'a' and 'd' positions of heptad repeats are shown in magenta. Full size image How does the complex subunit composition of CNG channels come about? The CNGA subunits contain a carboxy-terminal leucine zipper (CLZ) domain in the post-CNBD region ( Fig. 1a,b ) [8] . On the basis of the finding that the CLZ domain from CNGA3 forms homotypic trimers in solution, it was proposed that trimerization of this domain constrains the channel to contain three CNGA subunits [8] . Previously, it has been shown that point mutations in this domain decreased the proportion of heteromeric channels (relative to CNGA homomers) but did not alter the 3:1 stoichiometry of the heteromeric channels [20] . Here we test the role of the CLZ domain by measuring the subunit composition of CNGA1+CNGB1 channels when the CLZ domain in the CNGA1 subunit was deleted. Using electrophysiology and fluorescence measurements, we found that deletion of the CLZ domain relaxed the constrained subunit stoichiometry. This allowed more than one CNGB1 subunit in the channel and conferred novel pharmacological properties and cyclic nucleotide specificity. Using X-ray crystallography, we found that the CLZ domains of both CNGA1 and CNGA3 formed homotypic parallel 3-helix coiled-coil domains, consistent with their proposed role in regulating subunit assembly. Deletion of the CLZ domain affects cyclic nucleotide specificity To determine the role of the CLZ domain in controlling heteromeric assembly of CNGA1+CNGB1 channels, we first measured the functional effects of deleting the CLZ domain. CNG channels were expressed in Xenopus oocytes and studied using the inside–out configuration of the patch-clamp technique. Homomeric channels of CNGA1 subunits are efficiently activated by saturating cGMP, but poorly activated by saturating cAMP ( I cAMP / I cGMP =0.05±0.01, n =6) ( Fig. 2a , black is with 2.5 mM cGMP, red is with 16 mM cAMP). However, incorporation of a single CNGB1 subunit per tetramer confers a significant elevation in cAMP efficacy ( I cAMP / I cGMP =0.22±0.03, n =7) ( Fig. 2a ). The mechanism of the increased cAMP efficacy by the CNGB1 subunit is unknown but could involve either cAMP binding to CNGB1 or simply a more favourable opening transition with CNGB1 (or both). This increased efficacy is constant over a wide range of CNGB1 expression levels, indicating that the CNGB1 subunit incorporates into the channel with a fixed and tightly-regulated stoichiometry [15] . 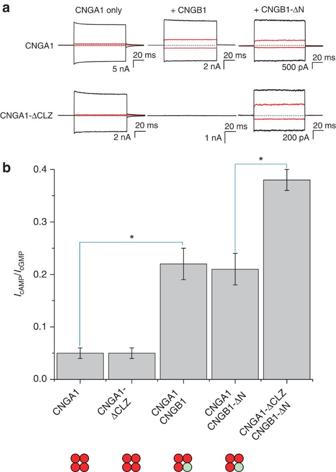Figure 2: Deletion of the CNGA1 CLZ domain increased the cAMP efficacy of heteromeric CNG channels. (a) Leak subtracted macroscopic current traces from inside–out patches in the presence of 2.5 mM cGMP (black) and 16 mM cAMP (red) in response to voltage pulses of −60 mV and +60 mV. Currents were recorded for CNGA1 only (top left), CNGA1-ΔCLZ only (bottom left), CNGA1+CNGB1 (top middle), CNGA1-ΔCLZ +CNGB1 (bottom middle), CNGA1+CNGB1-ΔN (top right), CNGA1-ΔCLZ +CNGB1-ΔN (bottom right). (b)IcAMP/IcGMPat +60 mV for each channel composition: CNGA1 (n=6), CNGA1-ΔCLZ (n=6), CNGA1+CNGB1 (n=7), CNGA1-ΔCLZ +CNGB1 (n=7), and CNGA1-ΔCLZ +CNGB1-ΔN (n=10). The expected subunit stoichiometry for each case is shown at the bottom. Data are plotted as mean±s.e.m. Asterisks denote statistically significant differences withP<0.01. Figure 2: Deletion of the CNGA1 CLZ domain increased the cAMP efficacy of heteromeric CNG channels. ( a ) Leak subtracted macroscopic current traces from inside–out patches in the presence of 2.5 mM cGMP (black) and 16 mM cAMP (red) in response to voltage pulses of −60 mV and +60 mV. Currents were recorded for CNGA1 only (top left), CNGA1-ΔCLZ only (bottom left), CNGA1+CNGB1 (top middle), CNGA1-ΔCLZ +CNGB1 (bottom middle), CNGA1+CNGB1-ΔN (top right), CNGA1-ΔCLZ +CNGB1-ΔN (bottom right). ( b ) I cAMP / I cGMP at +60 mV for each channel composition: CNGA1 ( n =6), CNGA1-ΔCLZ ( n =6), CNGA1+CNGB1 ( n =7), CNGA1-ΔCLZ +CNGB1 ( n =7), and CNGA1-ΔCLZ +CNGB1-ΔN ( n =10). The expected subunit stoichiometry for each case is shown at the bottom. Data are plotted as mean±s.e.m. Asterisks denote statistically significant differences with P <0.01. Full size image Previously, it has been shown that the amino-terminal region of the CNGB1 subunit interacts with the CLZ domain of the CNGA1 subunit and regulates trafficking of heteromeric channels [21] . To test for a possible role of this interaction in subunit assembly, we deleted the amino-terminal region (amino acids 2-765) of CNGB1 (CNGB1-ΔN). Co-expressing CNGA1 and CNGB1-ΔN produced robust currents with amplitude similar to that of CNGA1+CNGB1 (ref. 21 ). In addition, as shown in Figure 2a , deletion of the amino-terminal region of CNGB1 had no effect on the cAMP efficacy of the heteromeric channels ( I cAMP / I cGMP =0.21±0.03, n =7). These results suggest that the amino-terminal domain of CNGB1 is not required for the proper assembly of functional heteromeric channels. Next, we tested the effects of deletion of the CLZ domain (amino acids 609–693) of the CNGA1 subunit (CNGA1-ΔCLZ). Deletion of the CLZ domain had no effect on the expression or measured functional properties of CNGA1-ΔCLZ homomeric channels ( Fig. 2a ) [21] . However, it had a dramatic effect on expression and functional properties of CNGA1-ΔCLZ+ CNGB1 heteromeric channels. As shown previously, co-expression of CNGA1-ΔCLZ with CNGB1 at a typical 1:4 RNA ratio virtually eliminated all functional channel expression ( Fig. 2a ) [21] . This dominant negative effect may underlie one form of retinitis pigmentosa resulting from deletion of a portion of the CLZ domain in CNGA1 (refs 21 , 22 ) and suggests that the CNGA1-ΔCLZ channels are still interacting with CNGB1, perhaps in an uncontrolled manner. To recover functional expression of heteromeric channels, we co-injected CNGA1-ΔCLZ with CNGB1-ΔN containing a deletion of the trafficking signal in the amino-terminal region of CNGB1 (ref. 21 ). Even at an RNA ratio of 1:2 CNGA1-ΔCLZ:CNGB1-ΔN, the effect of the CLZ domain deletion on the heteromeric channels was striking. Co-expression of CNGA1-ΔCLZ and CNGB1-ΔN yielded channels with a highly elevated cAMP efficacy ( I cAMP / I cGMP =0.38±0.02, n =10) ( Fig. 2a ), significantly higher than CNGA1 homomeric channels and CNGA1+CNGB1 heteromeric channels ( Fig. 2b ). The elevated cAMP efficacy seen with the CLZ domain deletion in heteromeric channels, but not homomeric channels, suggests the possibility that CNGA1-ΔCLZ and CNGB1-ΔN form heteromeric channels with a novel stoichiometry, perhaps with more than one CNGB1 subunit per channel. Effects of deletion of the CLZ domain on L-cis-diltiazem block To further test for incorporation of multiple CNGB1 subunits on deletion of the CLZ domain, we measured the pharmacological properties of heteromeric channels. Although 100 μM L- cis -diltiazem is ineffective at blocking CNGA1 homomers, it potently blocks CNGA1+CNGB1 heteromers ( Fig. 3a , black is control, blue is 100 μM L- cis -diltiazem) [17] . The block is voltage dependent with a Hill slope of one, suggesting a pore-blocking mechanism ( Fig. 3a,b ). The CNGA1-ΔCLZ mutation had no effect on block of homomeric channels, and the CNGB1-ΔN mutation had no effect on block of heteromeric channels. Surprisingly, the block of CNGA1-ΔCLZ+CNGB1-ΔN heteromers was intermediate between CNGA1 (or CNGA1-ΔCLZ) homomers and CNGA1+CNGB1 (or CNGA1+ CNGB1-ΔN) heteromers ( Fig. 3a ). Previously, it was shown that heteromers formed with point mutations in the CLZ domain of CNGA3 exhibited intermediate block by L- cis -diltiazem because they formed mixtures of CNGA3 homomers and CNGA3+CNGB1 heteromers [20] . However, that was not the case here. As shown above, CNGA1-ΔCLZ+CNGB1-ΔN heteromers actually exhibit greater cAMP efficacy than either CNGA1 homomers or CNGA1+CNGB1 heteromers ( Fig. 2 ). Together, these results indicate the formation of a previously uncharacterized population of heteromeric CNG channel complexes. 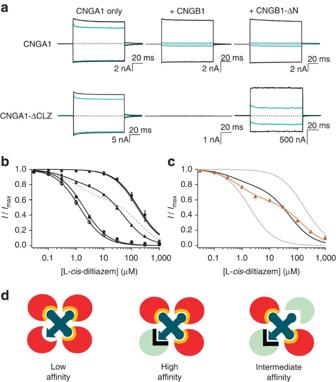Figure 3: Deletion of the CNGA1 CLZ domain confers intermediate L-cis-diltiazem block on heteromeric CNG channels. (a) cGMP-activated current traces from inside–out patches in the absence (black) and presence (blue) of 100 μM L-cis-diltiazem in response to voltage pulses of −60 mV and +60 mV. Currents were recorded for CNGA1 only (top left), CNGA1-ΔCLZ only (bottom left), CNGA1+CNGB1 (top middle), CNGA1-ΔCLZ +CNGB1 (bottom middle), CNGA1+CNGB1-ΔN (top right), and CNGA1-ΔCLZ +CNGB1-ΔN (bottom right). (b) Dose-response relations of L-cis-diltiazem block at +60 mV for CNGA1 only (n=5, filled squares), CNGA1-ΔCLZ only (n=6, open squares), CNGA1+CNGB1 (n=5, filled circles), CNGA1+CNGB1-ΔN (n=5, open circles), and CNGA1-ΔCLZ +CNGB1-ΔN (n=4, filled triangles). Data are plotted as mean±s.e.m. Data are fitted with a single Langmuir isotherm or the sum of two Langmuir isotherms (for CNGA1-ΔCLZ +CNGB1-ΔN). The dashed line shows the poor fit of CNGA1-ΔCLZ +CNGB1-ΔN with two Langmuir isotherms with affinities constrained to those of CNGA1-ΔCLZ only and CNGA1+CNGB1-ΔN. (c) Dose-response relation of L-cis-diltiazem block at +60 mV for CNGA1-ΔCLZ +CNGB1-ΔN at an RNA ratio of 1:1 (orange triangles) fitted with the sum of two Langmuir isotherms (orange line). Single Langmuir isotherms from CNGA1 only and CNGA1+CNGB1 are shown in grey and the sum of two Langmuir isotherms from CNGA1-ΔCLZ +CNGB1-ΔN at an RNA ratio of 1:2 is shown in black. (d) Cartoon depicting how interactions between a single molecule of L-cis-diltiazem (blue), and CNGA1 (red) and CNGB1 (green) subunits, could produce an intermediate affinity for channels containing multiple CNGB1 subunits. Figure 3: Deletion of the CNGA1 CLZ domain confers intermediate L- cis -diltiazem block on heteromeric CNG channels. ( a ) cGMP-activated current traces from inside–out patches in the absence (black) and presence (blue) of 100 μM L- cis -diltiazem in response to voltage pulses of −60 mV and +60 mV. Currents were recorded for CNGA1 only (top left), CNGA1-ΔCLZ only (bottom left), CNGA1+CNGB1 (top middle), CNGA1-ΔCLZ +CNGB1 (bottom middle), CNGA1+CNGB1-ΔN (top right), and CNGA1-ΔCLZ +CNGB1-ΔN (bottom right). ( b ) Dose-response relations of L- cis -diltiazem block at +60 mV for CNGA1 only ( n =5, filled squares), CNGA1-ΔCLZ only ( n =6, open squares), CNGA1+CNGB1 ( n =5, filled circles), CNGA1+CNGB1-ΔN ( n =5, open circles), and CNGA1-ΔCLZ +CNGB1-ΔN ( n =4, filled triangles). Data are plotted as mean±s.e.m. Data are fitted with a single Langmuir isotherm or the sum of two Langmuir isotherms (for CNGA1-ΔCLZ +CNGB1-ΔN). The dashed line shows the poor fit of CNGA1-ΔCLZ +CNGB1-ΔN with two Langmuir isotherms with affinities constrained to those of CNGA1-ΔCLZ only and CNGA1+CNGB1-ΔN. ( c ) Dose-response relation of L- cis -diltiazem block at +60 mV for CNGA1-ΔCLZ +CNGB1-ΔN at an RNA ratio of 1:1 (orange triangles) fitted with the sum of two Langmuir isotherms (orange line). Single Langmuir isotherms from CNGA1 only and CNGA1+CNGB1 are shown in grey and the sum of two Langmuir isotherms from CNGA1-ΔCLZ +CNGB1-ΔN at an RNA ratio of 1:2 is shown in black. ( d ) Cartoon depicting how interactions between a single molecule of L- cis -diltiazem (blue), and CNGA1 (red) and CNGB1 (green) subunits, could produce an intermediate affinity for channels containing multiple CNGB1 subunits. Full size image To unravel the cause of this intermediate block, we measured the dose-response relations for L- cis -diltiazem block at +60 mV. The dose-response relations for channels containing CLZ domains were well fit with a single Langmuir isotherm, suggesting a single population of channels ( Fig. 3b ). The block of CNGA1 and CNGA1-ΔCLZ homomers were similar and low affinity (K 1/2 =174±7.2 μM, n =5 and K 1/2 =164±8.2 μM, n =6, respectively), and the block of CNGA1+CNGB1 and CNGA1+ CNGB1-ΔN heteromers were similar and high affinity (K 1/2 =2.45±0.28 μM, n =5 and K 1/2 =1.40±0.21 μM, n =5, respectively) ( Fig. 3b ). The dose-response relation for block of CNGA1-ΔCLZ+CNGB1-ΔN heteromers, however, was not fit well by either a single Langmuir isotherm, nor by the sum of two Langmuir isotherms with affinities constrained to those of CNGA1 homomers and CNGA1+CNGB1 heteromers. Instead, fits to the sum of two Langmuir isotherms revealed a small high affinity component similar to that of CNGA1+CNGB1 channels (K 1/2 =0.56±0.09 μM, n =4), and a larger component with an affinity intermediate between that of CNGA1 homomers and CNGA1+CNGB1 heteromers (K 1/2 =50±5 μM, n =4) ( Fig. 3b ). These results suggest that the heteromers formed from CNGA1-ΔCLZ and CNGB1-ΔN are not a mixture of CNGA1 homomers and normal CNGA1+CNGB1 heteromers, but, instead, a mixture of normal 3:1 CNGA1+CNGB1 heteromers and novel CNGA1+CNGB1 heteromers. One intriguing possibility is that the novel heteromers formed without a CLZ domain contain multiple CNGB1 subunits. This would also suggest that whereas one CNGB1 subunit confers much greater L- cis -diltiazem affinity, extra CNGB1 subunits lower the L- cis -diltiazem affinity ( Fig. 3d ). This model predicts that lowering the relative amount of expressed CNGB1 subunits should actually increase the fraction of the high affinity component (due presumably to channels with the normal 3:1 CNGA1:CNGB1 stoichiometry), because a lower amount of CNGB1 should favour a subunit stoichiometry with fewer CNGB1 subunits. The results of such an experiment are shown in Figure 3c . Lowering the RNA co-injection ratio of CNGA1-ΔCLZ and CNGB1-ΔN from 1:2 to 1:1 significantly increased the fraction of the high affinity component from 0.21±0.01, n =3 to 0.40±0.01, n =4. In addition, the dose-response relation is now poorly fit by a sum of two Langmuir isotherms and is suggestive of a third component with an affinity similar to CNGA1 homomers. Together, these results suggest that deletion of the CLZ domain removes the constraint allowing only one CNGB1 subunit in the channel tetramer. This allows multiple CNGB1 subunits that confer higher efficacy for cAMP and (surprisingly) lower affinity for L- cis -diltiazem block ( Fig. 3d ). If channels containing three CNGB1 subunits were not functional or not trafficked properly to the plasma membrane, then this loss of controlled assembly could also explain the large dominant negative effect of CNGB1 subunits, when the CLZ domain is deleted from the CNGA1 subunit. Fluorescence measurements of multiple CNGB1 subunits To directly measure the presence of multiple CNGB1 subunits in the channel, we turned to an approach based on fluorescence resonance energy transfer (FRET) [23] . FRET reports the proximity of two fluorophores based on the efficiency of energy transfer between a donor fluorophore and an acceptor fluorophore. FRET can be detected by an enhanced emission of the acceptor fluorescence on excitation of the donor. Cyan fluorescent protein (eCFP) and yellow fluorescent protein (eYFP) are genetically-encoded donor and acceptor fluorophores, respectively, that can be fused to proteins of interest [24] . They exhibit 50% energy transfer at a distance of about 50 Å and measurable transfer up to 80 Å (ref. 25 ), making them ideally suited for measurements of subunit composition [7] . Previously it was shown that if CNGA1 subunits are fused to eCFP and eYFP (individually) and co-expressed with CNGB1 subunits in Xenopus oocytes, there was significant FRET for channels in the plasma membrane [7] . However, if CNGB1 subunits were fused to eCFP and eYFP and co-expressed with CNGA1 subunits, there was little or no FRET ( Fig. 4a ). These results revealed that heteromeric rod CNG channels in the plasma membrane contain multiple CNGA1 subunits but only a single CNGB1 subunit (3:1 stoichiometry). 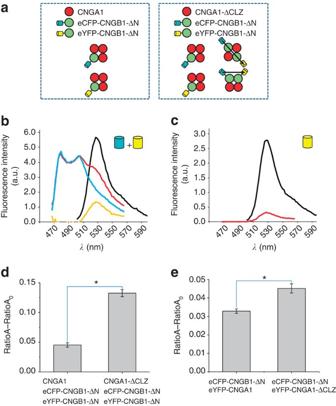Figure 4: FRET experiments reveal multiple CNGB1 subunits when the CNGA1 CLZ domain is deleted. (a) Predictions for FRET between eCFP-CNGB1-ΔN and eYFP-CNGB1-ΔN for channels containing just a single CNGB1 subunit (left) or possibly multiple subunits (right). Possibilities for FRET are shown by arrows. (b) Emission spectra ofXenopusoocytes expressing CNGA1-ΔCLZ with both eCFP-CNGB1-ΔN and eYFP-CNGB1-ΔN with 458 nm excitation (red) or 488 nm excitation (black). A scaled eCFP only excitation is shown in blue and extracted spectrum (difference between red and blue) is shown in yellow. Ratio A is the ratio of the yellow to the black spectrum. (c) Emission spectra of CNGA1-ΔCLZ+eYFP-CNGB1-ΔN coloured as in (b). Ratio Ao is the ratio of the red to the black spectrum. (d) Ratio A-Ratio Ao for FRET between CNGB1 subunits with (n=8) and without (n=6) the CLZ domain in the CNGA1 subunit. (e) Ratio A-Ratio Ao for FRET between CNGA1 and CNGB1 subunits with (n=6) and without (n=4) the CLZ domain in the CNGA1 subunit. Data are plotted as mean±s.e.m. Asterisks indicate statistically-significant differences, withP<0.05. Figure 4: FRET experiments reveal multiple CNGB1 subunits when the CNGA1 CLZ domain is deleted. ( a ) Predictions for FRET between eCFP-CNGB1-ΔN and eYFP-CNGB1-ΔN for channels containing just a single CNGB1 subunit (left) or possibly multiple subunits (right). Possibilities for FRET are shown by arrows. ( b ) Emission spectra of Xenopus oocytes expressing CNGA1-ΔCLZ with both eCFP-CNGB1-ΔN and eYFP-CNGB1-ΔN with 458 nm excitation (red) or 488 nm excitation (black). A scaled eCFP only excitation is shown in blue and extracted spectrum (difference between red and blue) is shown in yellow. Ratio A is the ratio of the yellow to the black spectrum. ( c ) Emission spectra of CNGA1-ΔCLZ+eYFP-CNGB1-ΔN coloured as in ( b ). Ratio Ao is the ratio of the red to the black spectrum. ( d ) Ratio A-Ratio Ao for FRET between CNGB1 subunits with ( n =8) and without ( n =6) the CLZ domain in the CNGA1 subunit. ( e ) Ratio A-Ratio Ao for FRET between CNGA1 and CNGB1 subunits with ( n =6) and without ( n =4) the CLZ domain in the CNGA1 subunit. Data are plotted as mean±s.e.m. Asterisks indicate statistically-significant differences, with P <0.05. Full size image We performed a similar experiment to determine if deletion of the CLZ domain permitted incorporation of multiple CNGB1 subunits into the heteromeric channels. If there are multiple CNGB1 subunits in the heteromeric channels, then we should observe FRET between CNGB1 subunits when fused to eCFP and eYFP and co-expressed with CNGA1-ΔCLZ subunits ( Fig. 4a ). For these experiments, we fused eCFP and eYFP (individually) to the amino-terminal end of CNGB1-ΔN (eCFP- CNGB1-ΔN and eYFP- CNGB1-ΔN respectively). The eCFP and eYFP fusion constructs exhibited functional properties indistinguishable from their non-fusion counterparts (data not shown). As the amino-terminal region is deleted in this subunit, the fluorescent proteins should be near the inner leaflet of the membrane, close to the S1 transmembrane segment. Based on the structure of the related Kv1.2 channel [26] , two fluorescent proteins in the same channel should be about 56 Å apart (assuming they are in adjacent subunits) or 79 Å apart (assuming they are in nonadjacent subunits). Representative results from co-expression of CNGA1-ΔCLZ with eCFP- CNGB1-ΔN and eYFP- CNGB1-ΔN are shown in Figure 4b . FRET was measured from the sensitized emission of the acceptor using fluorescence spectra [23] . The fluorescence emission spectra from channels in or near the plasma membrane of live Xenopus oocytes were measured with confocal microscopy. Excitation of eCFP with a 458 nm laser produced a complex emission spectrum (red trace) with both eCFP and eYFP emission components. The eYFP component (orange trace) was extracted by subtracting off a scaled emission spectrum from eCFP alone (blue trace). This extracted spectrum contains eYFP emission from both FRET and direct excitation of eYFP by 458 nm light. To isolate the component due to FRET, the fractional excitation of eYFP by 458 nm light relative to 488 nm light (Ratio Ao) ( Fig. 4c , Methods) was subtracted off the corresponding fractional excitation for eCFP and eYFP-containing channels (Ratio A). Ratio A-Ratio Ao is directly proportional to the FRET efficiency [23] . As shown in Figure 4d , Ratio A-Ratio Ao was significantly larger with CNGA1-ΔCLZ than with CNGA1, when the CNGA1 subunit was coexpressed with fluorescent CNGB1. These results directly demonstrate that deletion of the CLZ domain caused multiple CNGB1 subunits to assemble. A possible alternative explanation for the FRET seen between CNGB1 subunits with deletion of the CNGA1 CLZ domain is that the CNGB1 subunits are forming homomeric channels at low levels. Indeed, the fluorescence is considerably dimmer with co-expression of CNGA1-ΔCLZ than with CNGA1. Previously, however, it has been shown that, in the absence of CNGA1, CNGB1 subunits do not form functional homomeric channels and are only very weakly expressed in the plasma membrane [9] , [17] . Similarly, we found that, in the absence of a CNGA1 subunit, both CNGB1 and CNGB1-ΔN did not produce detectable currents and are poorly expressed in the plasma membrane ( Supplementary Fig. S1 ). In addition, it was shown previously that the CNGB1 subunits expressed alone do not exhibit appreciable FRET [9] . This makes it unlikely that the increased FRET seen between CNGB1 subunits with deletion of the CNGA1 CLZ domain is from CNGB1 subunits forming homomeric channels. Nevertheless, to prove that multiple CNGB1 subunits are co-assembled with CNGA1-ΔCLZ subunits, we examined the FRET between CNGA and CNGB subunits. For acceptor sensitization, the apparent FRET efficiency increases as the donor-to-acceptor ratio increases [27] . Therefore, if the donor fluorophore (eCFP) was fused to the CNGB subunit and the acceptor fluorophore (eYFP) was fused to the CNGA subunit, then an increase in apparent FRET should be seen if multiple CNGB1 subunits assembled in the channel complex ( Supplementary Fig. S2 ). Indeed, the results show a significant increase in FRET between eCFP-CNGB1-ΔN and eYFP-CNGA1-ΔCLZ compared with eYFP-CNGA1 ( Fig. 4e ). These results indicate that multiple CNGB1 subunits are co-assembling with CNGA1-ΔCLZ subunits. Overall, it is clear that deletion of the CLZ domain relaxes the 3:1 constraint on subunit assembly. The CLZ domains of CNGA1 and CNGA3 form trimers in solution The above results suggest that the CLZ domain has an important role in constraining the stoichiometry of rod CNG channels to 3:1 CNGA1:CNGB1 subunits. Previously, it has been shown that a protein fragment containing the CLZ domain from cone CNGA3 forms homotypic trimers in solution [8] . To determine whether the CLZ domain from CNGA1 would also form trimers, and to localize the region involved, we screened a number of carboxy-terminal fragments of both CNGA1 and CNGA3 using fluorescence-detection size-exclusion chromatography (FSEC) ( Supplementary Fig. S3 ) [28] . The protein fragments were expressed in bacteria as N-terminal (NGFP) or C-terminal (CGFP) fusions to GFP. After cell lysis, the crude supernatant was then loaded on a size-exclusion chromatography system with an inline fluorescence detector. All the expressing fragments that contained the CLZ domain showed an appreciable component that eluted at 13 mL, consistent with the formation of a trimer ( Fig. 5a ). To verify the composition of the high molecular weight component, samples of the purified protein, following cleavage of GFP, were analysed by light scattering size-exclusion chromatography (LS-SEC) ( Fig. 5b ) [29] , [30] . For both CNGA1 and CNGA3, the molecular weights determined from LS-SEC were within about 1% of the predicted molecular weights for a trimer ( Table 1 ). Similar results with smaller fragments revealed a minimal fragment, corresponding to the CLZ domain, that formed trimers in both CNGA1 (amino acids 621–667) and CNGA3 (626–672) subunits. 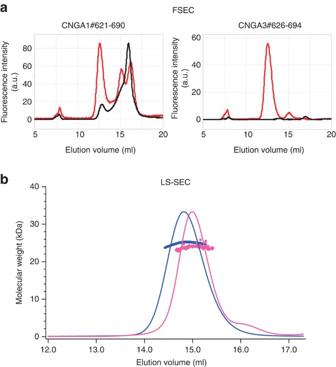Figure 5: Size-exclusion chromatography and light scattering reveal the CLZ domains from CNGA1 and CNGA3 form trimers. (a) FSEC results of CNGA1#621–690 (left) and CNGA3#626–694 (right) as N-terminal (red) and C-terminal (black) fusions to GFP. The peaks eluting at 13 mL are the predicted size for a trimer of the fusion proteins. (b) LS-SEC results of CNGA1#621–690 (blue) and CNGA3#626–694 (magenta). The smooth traces show the elution of the protein (ultraviolet absorbance) and the data points show the measured molecular weight (left axis). Figure 5: Size-exclusion chromatography and light scattering reveal the CLZ domains from CNGA1 and CNGA3 form trimers. ( a ) FSEC results of CNGA1#621–690 (left) and CNGA3#626–694 (right) as N-terminal (red) and C-terminal (black) fusions to GFP. The peaks eluting at 13 mL are the predicted size for a trimer of the fusion proteins. ( b ) LS-SEC results of CNGA1#621–690 (blue) and CNGA3#626–694 (magenta). The smooth traces show the elution of the protein (ultraviolet absorbance) and the data points show the measured molecular weight (left axis). Full size image Table 1 Summary of LS-SEC results. Full size table X-ray crystallography reveals a three helix coiled-coil domain The sequence of the CLZ domain exhibits periodic heptad repeats (a-b-c-d-e-f-g) n in which the 'a' and 'd' positions are hydrophobic residues ( Fig. 1b ) [8] . This motif is characteristic of coiled-coil domains [31] , [32] . There are two noncontiguous heptad repeat regions in each sequence; the first has three repeats and the second has two repeats. The two regions are out of register, with the 'a' position of the first region becoming the 'd' position of the second region. While the presence of heptad repeats is fairly indicative of coiled-coil domains, it is difficult to determine from the sequence alone the oligomeric state, parallel versus antiparallel arrangement, and details of the coiled-coil packing and surface architecture [32] . These properties have direct bearing on the mechanism of assembly, the interpretation of mutations, and the interaction with other proteins or domains. For these reasons, we were interested in obtaining the high-resolution structure of the CLZ domains. We have solved the high-resolution X-ray crystal structures of the CLZ domains of both CNGA1 and CNGA3. The proteins were expressed and purified from bacterial cell lysates and crystallized under vapour diffusion. Crystals of CNGA1#621–690 grew in space group P2 1 2 1 2 1 with three molecules in the asymmetric unit and diffracted to 2.14 Å. The structure of CNGA1#621–690 was solved using molecular replacement with the structure of HIV gp41 N-trimer pocket region [33] (3L36) as a search probe ( Supplementary Table S1 ). The structure of CNGA3#626–672 in space group P12 1 1 was solved to 1.9 Å using molecular replacement with the structure of SARS virus S2 protein [34] (1ZVB) as a search probe ( Supplementary Table S1 ). The structures of both CNGA1#621–690 and CNGA3#626–672 consisted of long (65 Å) parallel three-helix coiled-coil domains ( Fig. 6 ). The sequence beyond the CLZ domain in CNGA1 (amino acids 665–675 for chain A; 665–676 for chain B; and 665–670 for chain C) flared outward and was partially involved in crystal packing interactions ( Supplementary Fig. S4 ). In addition, the CNGA1#621–690 structure contained two bound heavy atoms per trimer with an electron density greater than 10 sigma ( Fig. 6 ; Supplementary Fig. S5 ). These heavy atoms were coordinated by acidic residues (E629 and D633 for the proximal site, and E671 and E623 for the distal ion) at the interface between different trimers in the crystal and, therefore, are presumed to be non-physiological ( Supplementary Fig. S5 ). They are likely to be Zn 2+ ions because of their coordination and the requirement for Zn 2+ in the crystallization solution to produce crystals. 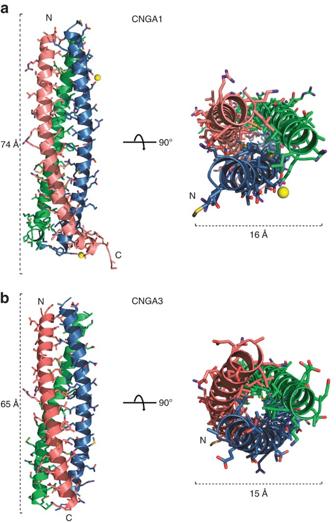Figure 6: Structure of the trimeric coiled-coil CNGA CLZ complexes. Ribbon representation of the trimeric coiled-coil structures of CNGA1#621–690 (a) and CNGA3#626–672 (b). Each complex is shown from a side (left) and top (right) perspective (top, N-terminus; bottom, C-terminus). The metal ions coordinated by the glutamate and aspartate residues at two sites in CNGA1#621–690 are shown as yellow spheres. Figure 6: Structure of the trimeric coiled-coil CNGA CLZ complexes. Ribbon representation of the trimeric coiled-coil structures of CNGA1#621–690 ( a ) and CNGA3#626–672 ( b ). Each complex is shown from a side (left) and top (right) perspective (top, N-terminus; bottom, C-terminus). The metal ions coordinated by the glutamate and aspartate residues at two sites in CNGA1#621–690 are shown as yellow spheres. Full size image The packing of the coiled-coil domains followed the characteristic 'knobs into holes' arrangement with the 'a' and 'd' positions forming alternating layers of the hydrophobic core of the coiled coil ( Fig. 7 ) [32] , [35] . The two noncontiguous heptad repeat regions assembled into a single continuous coiled coil. Interestingly, the CNGA1 and CNGA3 structures differed in the length of the two heptad repeat regions. For CNGA1, the first region contained 3 heptad repeats and the second contained 3.5 repeats ( Fig. 7b ). For CNGA3 the first region contained 4 heptad repeats and the second contained 2.5 repeats ( Fig. 7c ). The difference appears to be the substitution of an isoleucine for a leucine after the third heptad repeat in CNGA1 ( Fig. 1b ). 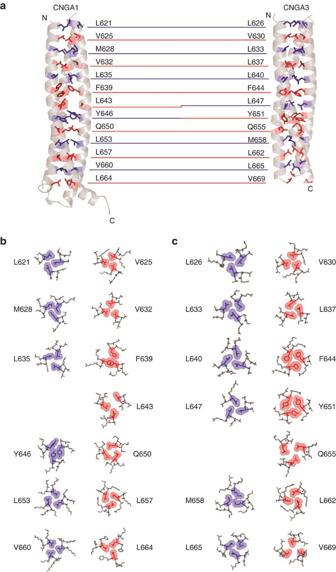Figure 7: Analysis of the hydrophobic packing in CNGA1 and CNGA3 CLZ domains. (a) Hydrophobic layers of CNGA1#621–690 (left) and CNGA3#626–672 (right). Side chains are depicted for the 'a' (red) and 'd' (blue) positions of the coiled coils. (b,c) Packing geometry for the 'a' (red) and 'd' (blue) positions of CNGA1#621–690 (b) and CNGA3#626–672 (c). Figure 7: Analysis of the hydrophobic packing in CNGA1 and CNGA3 CLZ domains. ( a ) Hydrophobic layers of CNGA1#621–690 (left) and CNGA3#626–672 (right). Side chains are depicted for the 'a' (red) and 'd' (blue) positions of the coiled coils. ( b , c ) Packing geometry for the 'a' (red) and 'd' (blue) positions of CNGA1#621–690 ( b ) and CNGA3#626–672 ( c ). Full size image Although the structures of CNGA1 and CNGA3 were generally similar, they were not identical. As stated above, different residue positions were used in the helical packing between the two heptad repeat regions in the sequence. In addition, the supercoiling was different between CNGA1 and CNGA3, with a somewhat longer pitch for CNGA1 (181 Å) than for CNGA3 (149 Å) ( Supplementary Table S2 ). These differences were also reflected in the structural alignments of the individual subunits of CNGA1 and CNGA3 (rmsd of Cα ranging from 0.87 Å to 2.0 Å). These differences in structure, however, do not have any known functional consequences. The results from the above experiments, and those of others, suggest a molecular mechanism for the controlled assembly of rod CNG channels with a 3:1 stoichiometry of CNGA1:CNGB1 subunits ( Fig. 8a ) [6] , [7] , [8] , [9] , [20] . In this mechanism, the CNGA1 subunits initially assemble into trimers through homotypic association of their carboxy-terminal CLZ domains into a parallel three helix coiled coil. Subsequently, a CNGB1 subunit, if present, is preferentially incorporated into the remaining slot of the channel tetramer because of a high affinity association with CNGA1 subunits. This mechanism incorporates aspects of two previous models for heteromeric assembly of CNG channels: initial assembly of CNGA1 trimers [8] , and high affinity association between CNGA1 and CNGB1 subunits [9] , [21] . The trimerization of the CLZ domain imposes the constraint that the channels contain at least three CNGA1 subunits, whereas the high affinity association between CNGA1 and CNGB1 assures that the fourth subunit is CNGB1. In support of this mechanism, we showed with electrophysiology and fluorescence that deletion of the CLZ domain in CNGA1 causes multiple CNGB1 subunits to incorporate into the heteromeric CNG channel. Furthermore, with X-ray crystallography we showed that there is a trimerization of the CLZ domain for both CNGA1 and CNGA3 ( Fig. 5 ) that results from the formation of a parallel three helix coiled coil ( Fig. 6 ). 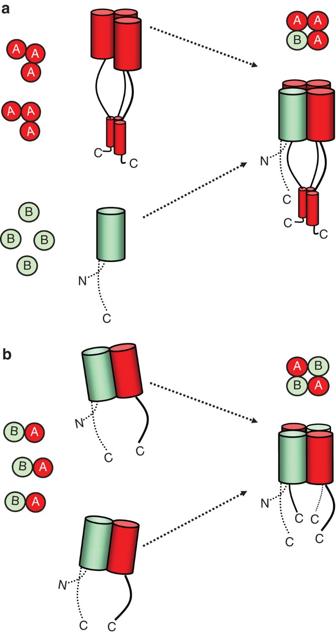Figure 8: Mechanism for the controlled assembly of heteromeric rod CNG channels. (a) The CNGA1 subunits (red) initially assemble into trimers through homotypic association of their carboxy-terminal CLZ domains into a parallel three helix coiled coil. Subsequently, a CNGB1 subunit (green), if present, is preferentially incorporated into the remaining slot of the channel tetramer due to a high affinity association with CNGA1 subunits. (b) Deletion of the CLZ domain in CNGA1 allows CNGA1 subunits to assemble with CNGB1 subunits. This produces channels with multiple CNGB1 subunits and a large dominant negative effect of CNGB1. Figure 8: Mechanism for the controlled assembly of heteromeric rod CNG channels. ( a ) The CNGA1 subunits (red) initially assemble into trimers through homotypic association of their carboxy-terminal CLZ domains into a parallel three helix coiled coil. Subsequently, a CNGB1 subunit (green), if present, is preferentially incorporated into the remaining slot of the channel tetramer due to a high affinity association with CNGA1 subunits. ( b ) Deletion of the CLZ domain in CNGA1 allows CNGA1 subunits to assemble with CNGB1 subunits. This produces channels with multiple CNGB1 subunits and a large dominant negative effect of CNGB1. Full size image In an elegant series of experiments, Yau and co-workers have proposed a mechanism for 3:1 CNGA:CNGB assembly that involves initial assembly of CNGA trimers [8] . They show that other three helix coiled coils, but not two helix or four helix coiled coils, could substitute for the CLZ domain of CNGA channels to reproduce normal heteromeric channel function and expression [20] . However, whereas we found that deletion of the CLZ domain causes an increase in CNGB1 incorporation in the channels, they showed that mutations in the CLZ domain decreased the incorporation of CNGB1 subunits [20] . Their results were explained by an assembly model where excess CNGA1 monomers outcompete CNGB1 monomers for channel incorporation. Instead, we propose that CNGB1 monomers outcompete CNGA1 monomers for channel incorporation owing to a high affinity association of CNGA1 and CNGB1 subunits. A high affinity association between CNGA and CNGB subunits has been previously proposed to explain the dependence of the CNGA:CNGB ratio in the surface membrane as a function of the ratio of their RNAs injected into the oocyte [9] . A high affinity association of CNGA1 and CNGB1 subunits also explains the large dominant negative effect of CNGB1 on deletion of the CLZ domain in CNGA1 ( Fig. 2a ) [21] . When the CLZ domain is deleted, the CNGA1 subunits preferentially interact with CNGB1 subunits, resulting in channels with multiple CNGB1 subunits that are not as efficiently expressed in the plasma membrane ( Fig. 8b ). This defect has been proposed to underlie one form of inherited retinitis pigmentosa resulting from deletion of the last two heptad repeats of the CLZ domain of CNGA1 (refs 21 , 22 ). Previously, it has been shown that deletion of the amino-terminal region of CNGB1 could partially restore expression of these CNGA1-ΔCLZ-containing channels [21] , suggesting that the amino-terminal region of CNGB1 might be involved in the high-affinity association between CNGA1 and CNGB1 subunits. Alternatively, the amino-terminal region of CNGB1 could contain a trafficking signal for incorrectly assembled heteromeric CNG channels [21] . This trafficking signal could provide a mechanism for error-correction where channels with more than one CNGB1 subunit are either poorly trafficked to the plasma membrane or rapidly removed from the membrane. Beyond channel assembly, the CLZ coiled-coil domain may also serve as a scaffold for interactions with other proteins. Previously, it has been shown that the calmodulin binding site in the amino-terminal region of CNGB1 directly interacts with the CLZ domain of CNGA1 (refs 36 , 37 ). Furthermore, Ca 2+ -calmodulin disrupts this interaction resulting in separation of the amino-terminal region of CNGB1 from the carboxy-terminal region of CNGA1 (ref. 38 ). Also, the CLZ coiled-coil domain may be an important site of interaction for protein complexes that regulate channel activity, as has been proposed for Kv7 channels [39] , [40] , [41] . Although the subunit stoichiometry of the rod CNG channel has been well established, the stoichiometry of the cone CNG channel is still uncertain. Whereas some studies have suggested it also has a 3:1 stoichiometry of CNGA3:CNGB3, others have suggested a 2:2 stoichiometry [8] , [10] . Here we find that the CLZ domain of CNGA3 forms a parallel three helix coiled coil that is similar to that of CNGA1. This suggests that the stoichiometry and mechanism of assembly for the cone CNG channel will be similar to that of the rod CNG channel. In addition, it has been shown that other three helix coiled-coil domains can substitute for the CLZ domain in cone CNG channels, but two and four helix coiled-coil domains cannot [20] . Interestingly, the olfactory CNG channel has a stoichiometry of 2:1:1 CNGA2:CNGA4:CNGB1b [9] . Both the CNGA2 and CNGA4 subunits have a CLZ domain ( Fig. 1b ). It remains to be determined whether the 2:1:1 stoichiometry comes about from a heterotypic three helix coiled coil of the CNGA2 and CNGA4 subunits, or from other intersubunit interactions such as seen at the level of the C-linker regions in the related hyperpolarization-activated cyclic nucleotide-gated channels [19] . In addition, the 3:1 stoichiometry of the TRPP2/PKD1 complex has recently been proposed to involve a trimeric coiled-coil domain in the carboxy-terminal region of TRPP2 (ref. 42 ), suggesting that the assembly mechanism of CNG channels may extend to other distantly related proteins. Molecular biology The bovine CNGA1 complementary DNA used was described previously [43] , [44] and contains a C-terminal FLAG epitope (DYKDDYK). The bovine CNGB1 cDNA was a kind gift from Dr. R. Molday [14] and the human CNGA3 cDNA was a kind gift from Dr. K.W. Yau [45] . CNGA1-ΔCLZ (CNGA1-Δ609–693) and the CNGB1-ΔN (CNGB1-Δ2-765) were made as described [21] . CNGB1-ΔN had a further manipulation, where its internal Nco I restriction site was removed via silent mutation and re-inserted at the initial methionine codon using a PCR-based method. Improved monomeric versions of eCFP and eYFP (mCerulean and mCitrine) were employed in the generation of all fluorescent protein fusions with CNG subunits used for FRET experiments. cDNAs for mCerulean and mCitrine were kindly provided by Dr D Piston [46] and Dr RY Tsien [47] , respectively. All constructs were confirmed with fluorescence-based automated sequencing. cDNAs were subcloned into the high-expression pGEMHE vector [48] for expression in Xenopus oocytes. Vectors were linearized and complementary RNA (cRNA) was transcribed using the mMessage mMachine kit (Ambion). For co-injection experiments, relative amounts of RNA were quantified on agarose gels with a densitometric method. CNGA1 and CNGB1 were injected at an RNA ratio of 1:4 that has previously been shown to produce a pure population of heteromeric channels [15] . CNGA1-ΔCLZ and CNGB1-ΔN were injected at an RNA ratio of 1:2, and eCFP- CNGB1-ΔN and eYFP-CNGB1-ΔN were injected at an RNA ratio of 2:1. Electrophysiology Xenopus oocytes were microinjected with cRNA as previously described [49] . Cells were incubated at 16 °C for 5–8 days post-injection. Oocytes were patch clamped using the excised, inside–out configuration [50] with an Axopatch 200A patch-clamp amplifier (Axon Instruments) coupled to an ITC-16 AD converter (Instrutech). Data were recorded and analysed with Pulse (Instrutech) and further analysed offline with Igor (Wavemetrics). Currents were filtered at 2 kHz and sampled at 10 kHz. Recordings were made at room temperature ( ∼ 20 °C) using 0.25–0.75 MΩ glass pipettes. Following excision, patches were placed in saturating cGMP solution for a minimum of 25 min to ensure complete run-up [51] . Currents were recorded with voltage steps to +60 and −60 mV from a holding potential of 0 mV in the presence of saturating cGMP (2.5 mM) or saturating cAMP (16 mM). Leak currents recorded in the absence of cyclic nucleotide were subtracted. Bath and pipette solutions were identical and contained 130 mM NaCl, 0.2 mM EDTA, and 3 mM HEPES, pH 7.2. Ligand-containing solutions were identical to the bath solution but contained saturating cGMP or cAMP (2.5 mM and 16 mM, respectively). Internal solutions were applied with an RSC-100 solution changer (Molecular Kinetics). A 10 mM L- cis -diltiazem (BIOMOL) stock solution was made in 2.5 mM cGMP recording solution, then aliquotted and frozen at −20 °C. L- cis -diltiazem dilutions in saturating cGMP recording solution were prepared immediately before the collection of dose-response data. Dose-responses of L- cis -diltiazem block were constructed from the unblocked, leak-subtracted current at the end of a +60 mV pulse as a fraction of the current elicited in saturating cGMP, with no L- cis -diltiazem present. Dose-response relations were fit with either a single Langmuir isotherm: or the sum of two Langmuir isotherms: where K 1/2 is the apparent affinity and X is the fraction of the high affinity component (K a 1/2 ) relative to the low affinity component (K b 1/2 ). Spectral FRET method For FRET experiments, fluorescence images were collected using a X20 objective from the animal pole of oocytes with a confocal microscope (Leica SP1) using laser excitation at 458 nm and 488 nm. Regions of interest were drawn by hand in MetaMorph (Molecular Devices), and background fluorescence was quantified from the blank area inside the cell and subtracted ( Supplementary Fig. S6 ). The pinhole was adjusted so that the brightest cells were within the linear range of the detector with a maximum pinhole setting of 1 Airy unit. Data from cells with very dim fluorescent signals were discarded. Emission spectra were constructed over a range of wavelengths with an emission window of 2 nm. Spectra closely resembled the published spectra [46] , [47] , suggesting that the fluorescent properties of these fluorescent protein variants are retained despite their incorporation into fusion proteins. FRET calculations were made using the spectral FRET method, as previously described [7] , [9] , [23] . Protein biochemistry Four different CLZ containing constructs of varying lengths were generated for both CNGA1 and CNGA3 ( Supplementary Fig. 3 ). Each of these eight constructs was subcloned into two bacterial expression vectors, pNGFP_BC and pCGFP_BC (kindly provided by Dr. E. Gouaux), creating amino-terminal and carboxy-terminal GFP fusion proteins respectively. Each of these 16 constructs was screened by FSEC as previously described [28] . Briefly, 5 ml bacterial cultures were induced, spun down, and resuspended in 800 μl of 150 mM KCl, 30 mM HEPES, pH 7.5 containing 2.5 μg ml −1 DNAse and cOmplete protease inhibitor tablets (Roche). The cells were lysed with a probe sonicator; the lysate was cleared by centrifugation (1,700× g for 30 min); and 100 μl of the supernatant was loaded on a Superdex 200 10/300 GL column (GE Healthcare) mounted on an FPLC system with a fluorescence detector set for detection of GFP fluorescence. Four candidates from the FSEC screen (CNGA1#621–690, CNGA1#621–667, CNGA3#626–694, and CNGA3#626–672) were subjected to further analysis. For large scale protein preparations, the CNGA1 and CNGA3 channel fragments were subcloned into the pETGQ and pETM11 vectors, respectively, creating amino-terminal poly-His fusion proteins. For the CNGA3#626–672 construct, the Nco I site at the amino terminus was deleted using PCR-based methods. Two litre bacterial cultures were grown to mid-log phase and induced with 1 mM IPTG overnight at 18 °C. The cultures were spun down and resuspended in 150 mM KCl, 30 mM HEPES, pH 7.5 containing 1 mM AEBSF, 2.5 μg ml −1 DNAse and cOmplete protease inhibitor tablets (Roche). Cells were lysed with an EmulsiFlex C-5 homogenizer (Avestin), and the lysate was cleared by centrifugation at 131,000× g for 45 min at 4 °C. The proteins were then purified on a Ni 2+ affinity resin column (HisTrap HP, GE Healthcare). The octahistidine tag was removed by thrombin or TEV cleavage, and the proteins were further purified on an anion or cation exchange column (HiTrap Q HP or HiTrap SP FF, GE Healthcare) and concentrated. Two of the samples mentioned above (CNGA1#621–690, CNGA3#626–694) were submitted to the Biophysics Resource of the W.M. Keck Biotechnology Facility at Yale University (New Haven, CT) for LS-SEC analysis. The samples were run on a Superdex 200 10/300 GL column (GE Healthcare) in 150 mM NaCl, 20 μM EDTA, 50 mM Tris–HCL, pH 8.0 (CNGA1#621–690) or 150 mM KCl, 30 mM HEPES, pH 7.5 (CNGA3#626–694). The molecular weight was determined by solving the equation that relates the excess scattered light, measured at several angles, to the concentration of solute and the weight-average molar mass using the ASTRA program [30] . X-ray crystallography Crystals were grown by the sitting drop, vapour diffusion method at 20°C. Crystals of CNGA1#621–690 grew using a 1:1 mixture of protein and reservoir solution containing 18.2% (w/v) PEG 3350, 45 mM Zn 2+ acetate, 9 mM CoCl 2 . These conditions produced crystals within 8 days with space group P2 1 2 1 2 1 that diffracted to a resolution of 2.14 Å. Crystals of CNGA3#626–672 grew using a 1:1 mixture of protein and reservoir solution containing 20% (w/v) PEG 3350, 200 mM K + acetate. These conditions produced crystals within 1 day with space group P12 1 1 that diffracted to a resolution of 1.9 Å. For diffraction data collection, crystals were immersed in liquid nitrogen after cryoprotection in 20% glycerol. Data were collected at 110 °K on beamline 8.2.1 at the Advanced Light Source (Lawrence Berkeley National Laboratory, Berkeley). Integration, scaling and merging of the diffraction data were done with the Mosflm program [52] . The structures were solved by molecular replacement using the programs Phaser [53] and Phenix [54] . For CNGA1, the structure of HIV gp41 N-trimer pocket region [33] (3L36) was used as a search probe. For CNGA3, the structure of SARS virus S2 protein [34] (1ZVB) was used as a search probe. Molecular models were rebuilt using ARP/wARP (ref. 55 ) (CNGA1) or the Phenix software suite [54] (CNGA3). Structure refinement and validation were performed using the Phenix software suite [54] and the program Coot [56] using Fo – Fc ′omit′ maps. Based on the Ramachandran plot, the percent of amino acids in favoured/allowed/disallowed conformations were 99.37/0.63/0.0 for CNGA1 and 100.00/0.0/0.0 for CNGA3. The coiled-coil parameters were analysed by the program TWISTER [57] . Statistical analysis Data parameters were plotted as mean±s.e.m. Student's test was used to determine significance at P <0.05. Acccession codes: The structures of CNGA1#621-690 and CNGA3#626-672 have been deposited in the Protein Data Bank under ID codes 3SWF and 3SWY . How to cite this article: Shuart, N. G. et al . Molecular mechanism for 3:1 subunit stoichiometry of rod cyclic nucleotide-gated ion channels. Nat. Commun. 2:457 doi: 10.1038/ncomms1466 (2011).